Coexistent ARID1A–PIK3CA mutations promote ovarian clear-cell tumorigenesis through pro-tumorigenic inflammatory cytokine signalling Ovarian clear-cell carcinoma (OCCC) is an aggressive form of ovarian cancer with high ARID1A mutation rates. Here we present a mutant mouse model of OCCC. We find that ARID1A inactivation is not sufficient for tumour formation, but requires concurrent activation of the phosphoinositide 3-kinase catalytic subunit, PIK3CA. Remarkably, the mice develop highly penetrant tumours with OCCC-like histopathology, culminating in haemorrhagic ascites and a median survival period of 7.5 weeks. Therapeutic treatment with the pan-PI3K inhibitor, BKM120, prolongs mouse survival by inhibiting the tumour cell growth. Cross-species gene expression comparisons support a role for IL-6 inflammatory cytokine signalling in OCCC pathogenesis. We further show that ARID1A and PIK3CA mutations cooperate to promote tumour growth through sustained IL-6 overproduction. Our findings establish an epistatic relationship between SWI/SNF chromatin remodelling and PI3K pathway mutations in OCCC and demonstrate that these pathways converge on pro-tumorigenic cytokine signalling. We propose that ARID1A protects against inflammation-driven tumorigenesis. Epithelial ovarian cancer (EOC) ranks as the fifth leading cause of cancer death among women [1] . EOC consists of four major histologic tumour subtypes (serous, clear-cell, endometrioid or mucinous) and originates from the coelomic epithelium, which is the precursor to the ovarian surface epithelium (OSE) and Müllerian ductal epithelium [2] . The salpinge or fallopian tube of the Müllerian epithelial anlage is the more definitive source of serous EOC [3] . Endometriotic explants originating from more distal sites in the Müllerian epithelial anlage may have some propensity to give rise to clear-cell or endometrioid EOC in humans, but this alternate mechanism of pathogenesis has not been thoroughly investigated [4] , [5] . In addition to the histologic feature, each EOC subtype can be further classified into two distinct groups based on the disease progression, metastatic potential and molecular signature, with low-grade serous, clear-cell, mucinous and endometrioid subtypes being classified as Type I tumours and the high-grade serous subtype as Type II tumours [6] . In general, Type I tumours account for up to 25% of EOCs, are genomically stable and have lower metastatic potential than Type II tumours, which constitute most of the remaining EOC cases [6] . In addition, KRAS , BRAF , PIK3CA , PTEN and CTNNB1 (β-CATENIN) mutations have historically been associated with Type I tumours at varying frequencies, whereas Type II tumours are largely defined by high-frequency TRP53 (p53) mutations and chromosome instability [6] , [7] , [8] . Therefore, EOC consists of a heterogeneous group of cancers, each with unique clinical challenges and biology. OCCC is the most common Type I tumour, accounting for 5–25% of all EOC cases, with incidence varying between populations [9] , [10] , [11] . Endometriosis is recognized as a significant risk factor for OCCC [12] , [13] , [14] . Among all EOC subtypes, OCCC has the worst prognosis if diagnosed at an advanced stage of disease because of poor response rates to platinum-based chemotherapy [9] , [10] , [15] , [16] . Consequently, survival rates for women with advanced stage OCCC are low [9] , [10] , [15] , [16] . Although OCCC is the second leading cause of death from ovarian cancer, the aetiology and pathogenesis of this devastating disease are poorly understood. Recent genome-sequencing efforts support a strong genetic contribution to OCCC aetiology based on the discovery of high-frequency (up to 50%) ARID1A tumour mutations [17] , [18] . ARID1A is also somatically mutated in another Type I EOC, endometrioid carcinoma and several other gynaecologic cancers, including uterine clear-cell and endometrioid carcinomas, cervical carcinoma and uterine carcinosarcoma [19] , [20] . Additional tumour-sequencing studies have detected recurrent ARID1A mutations in several non-gynaecologic cancers and, taken together, components of the SWI/SNF complex are mutated in at least 20% of human cancers [19] , [21] , [22] , [23] . ARID1A is a subunit within the SWI/SNF chromatin remodelling complex that facilitates target substrate recognition; however, its role in OCCC tumour initiation and progression has, yet, to be fully elucidated [24] . Genetically engineered mouse models offer the opportunity to investigate the contribution of genetic factors to EOC aetiology and pathogenesis [25] . In this regard, early research using mouse models of EOC established causative roles for coexistent mutations in PTEN and KRAS or PTEN and WNT/β-CATENIN pathways in endometrioid EOC [7] , [8] . Recently, Guan et al . [26] reported a mouse model of endometrioid EOC involving coexistent mutations in PTEN and ARID1A . In this study, we describe a new mouse model that genetically and histologically resembles human OCCC and functionally implicates coexistent ARID1A and PIK3CA mutations in cancer causation. We further provide new mechanistic insight into OCCC pathogenesis by establishing a functional link between coexistent ARID1A–PIK3CA mutations and interleukin-6 (IL-6) signalling. Generation of a novel Arid1a conditional allele To establish a functional role for ARID1A mutations in ovarian clear-cell tumorigenesis, we generated a novel Arid1a conditional allele ( Arid1a fl ) by inserting loxP sites flanking exons 5 and 6 in ARID1A ( Fig. 1a,b ). Arid1a-null embryos die around gastrulation and thus they are not amenable to efficient protein extraction [27] . In light of its early embryonic lethality, we monoalleliclly inactivated ARID1A in embryonic tissues (via Sox2Cre [28] ) to verify our Arid1a fl allele in the whole animal. Using this approach, we observed an expected 50% reduction in total protein from whole-embryo lysates ( Fig. 1c,d ). We next sought to inactivate ARID1A in the OSE. To do this, we employed the intrabursal AdCRE recombination system [7] , [29] . Efficient CRE-mediated genetic recombination was consistently observed in the OSE and outer epithelial layers of tissues confined to the bursal space ( Fig. 1f,h,i ). We performed a series of intrabursal AdCRE injections on two independent cohorts of Arid1a fl/fl mice ( n =42) and followed them for ~1 year. The mice remained tumour free with no significant changes in survival, other than age-related mortality, similar to the phenotypes reported by Guan et al . [26] ( Supplementary Fig. 1 ). The observation that ARID1A loss does not lead to tumour formation supports the notion that ARID1A mutations require additional mutational ‘hits’ in the OSE before tumorigenesis can ensue [26] . 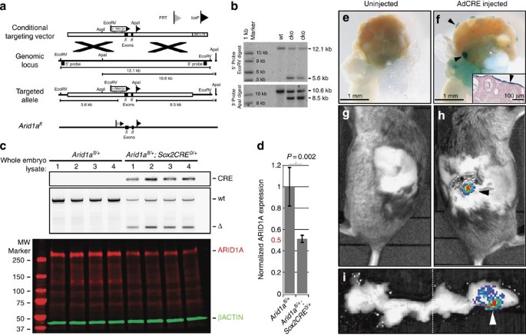Figure 1: A newArid1aconditional allele to explore ARID1A tumour-suppressor functionin vivo. (a) Targeting scheme to insert two loxP sites flanking exon 5 and 6 of mouse ARID1A. (b) Representative Southern blot showing properly targeted embryonic stem cell clones. Insertion of loxP sites generates 5.6 kb EcoRV and 8.5 kb ApaI genomic fragments. (c) PCR genotyping and quantitative, dual-colour fluorescent western blot of ARID1A (red) and βACTIN (green) protein expression in whole-embryo lysates from fourArid1afl/+and fourArid1afl/+;Sox2Cre0/+embryos. (d) Graph of quantitative western blot results depicting normalized protein levels. Significant differences based on the average normalized protein expression ±s.d. of four independent embryos were calculated using a two-tailed Student’st-test (Pvalues <0.05 were considered significant). (e,f) Representative LacZ-stained, control (uninjected) or intrabursal AdCRE-injected(Gt)Rosa26lacZovary showing patterns of CRE-mediated recombination in the OSE. (f, inset) Histological section of LacZ-stained AdCRE-injected(Gt)Rosa26lacZovary. (g–i) Live-luminescence overlaid whole-mount images of an intrabursal AdCRE-injected,(Gt)Rosa26luciferasefemale mouse. (i) Excised reproductive tract. Asterisks inhindicate wound staple. Figure 1: A new Arid1a conditional allele to explore ARID1A tumour-suppressor function in vivo . ( a ) Targeting scheme to insert two loxP sites flanking exon 5 and 6 of mouse ARID1A. ( b ) Representative Southern blot showing properly targeted embryonic stem cell clones. Insertion of loxP sites generates 5.6 kb EcoRV and 8.5 kb ApaI genomic fragments. ( c ) PCR genotyping and quantitative, dual-colour fluorescent western blot of ARID1A (red) and βACTIN (green) protein expression in whole-embryo lysates from four Arid1a fl/+ and four Arid1a fl/+ ;Sox2Cre 0/+ embryos. ( d ) Graph of quantitative western blot results depicting normalized protein levels. Significant differences based on the average normalized protein expression ±s.d. of four independent embryos were calculated using a two-tailed Student’s t -test ( P values <0.05 were considered significant). ( e , f ) Representative LacZ-stained, control (uninjected) or intrabursal AdCRE-injected (Gt)Rosa26lacZ ovary showing patterns of CRE-mediated recombination in the OSE. ( f , inset) Histological section of LacZ-stained AdCRE-injected (Gt)Rosa26lacZ ovary. ( g – i ) Live-luminescence overlaid whole-mount images of an intrabursal AdCRE-injected, (Gt)Rosa26luciferase female mouse. ( i ) Excised reproductive tract. Asterisks in h indicate wound staple. Full size image Coexistent ARID1A–PIK3CA mutations initiate ovarian cancer To explore this further, we focused on the cancer proto-oncogene, PIK3CA (Phosphatidylinositol-4,5-bisphosphate 3-kinase, catalytic subunit alpha or p110α), which also has high OCCC mutation rates [30] , [31] . Recently, coexistent ARID1A – PIK3CA mutations were reported in gastric cancer [32] . In addition, it has been observed that OCCC tumours harbouring PIK3CA mutations display a concomitant loss of ARID1A immunoreactivity, raising the possibility that ARID1A and PIK3CA mutations frequently co-occur in OCCC [33] . To understand the degree of mutational co-occurrence, we compared the incidence of ARID1A and/or PIK3CA mutations in available tumour data sets curated in The Cancer Genome Atlas (TCGA) to OCCC tumour-sequencing data [17] . We found that the majority of cancers carry genetic alterations in one of these genes; however, the rate of ARID1A – PIK3CA mutational co-occurrence (33%; P <0.05) is highest in OCCC ( Fig. 2a ). 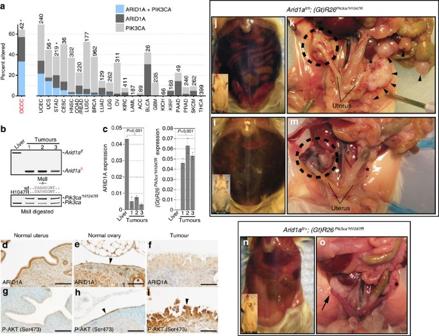Figure 2: Concurrent ARID1A loss and PIK3CA activation leads to ovarian tumorigenesis in the mouse. (a) Plot of ARID1A and PIK3CA alterations across available TCGA data sets. Mutation or co-mutation frequencies are expressed as a percentage of all tumour samples for each cancer. A Fisher’s exact test was used to calculate the significance of association between ARID1A and PIK3CA mutations (*Pvalue <0.05). (b) Genotyping scheme to detect CRE-deleted (Arid1aΔ) allele in tumour genomic DNA samples. RT–PCR was used to distinguishPIK3CAand transgenic(Gt)Rosa26Pik3ca*H1047Rtranscripts in tumour RNA samples. The H1047R mutation in(Gt)Rosa26Pik3ca*H1047Rprotects against MslI digest of amplified tumour cDNA. (c) ARID1A loss or(Gt)Rosa26Pik3ca*H1047Rtranscripts were detected in tumour RNA samples by RT–PCR. Significant differences based on the average normalized mRNA expression ±s.d. between replicates of a control liver sample and replicates of three independent tumour samples were calculated using a two-tailed Student’st-test (Pvalues <0.05 were considered significant). (d,e) ARID1A expression is observed in cells throughout the normal uterus and ovary by IHC. (e) ARID1A is expressed in the OSE of normal ovaries (arrowhead). (f) ARID1A expression is not observed in the tumours. (g) P-AKT S473 levels are low in the normal uterus. (h,i) P-AKT S473 in the normal ovary is highest in the OSE (h, arrowhead) and these levels are greatly increased in ovarian tumours (i, arrowhead). Asterisk inedenotes an oocyte. All sections processed for IHC were lightly counterstained with methyl green. (j,k) MorbidArid1afl/fl;(Gt)Rosa26Pik3ca*H1047Rmouse at killing with haemorrhagic ascites (inset), primary ovarian tumour of moderate size and bilateral tumour metastases (arrowheads). (l,m) MorbidArid1afl/fl;(Gt)Rosa26Pik3ca*H1047Rmouse at killing with haemorrhagic ascites (inset), large primary ovarian tumour and no visible metastases. The mice shown inj–mwere killed at 7 and 9 weeks post AdCRE, respectively, because of visible ascitic fluid burden. (n,o)Arid1afl/+;(Gt)Rosa26Pik3ca*H1047Rmice at 11 weeks post AdCRE showing no evidence for tumour formation. Ink,m, dashed circles indicate primary ovarian tumour on injected ovary. Inn, arrows denote the AdCRE-injected ovary. Ink,m,o, asterisks denote the uninjected, control ovary. ACC, adrenocortical carcinoma; BLCA, bladder urothelial carcinoma; BRCA, breast invasive carcinoma; CESC, cervical squamous cell carcinoma and endocervical adenocarcinoma; COAD/READ, colon and rectum adenocarcinoma; GBM, glioblastoma multiforme; HNSC, head and neck squamous cell carcinoma; KICH, kidney chromophobe; KIRC, kidney renal clear-cell carcinoma; KIRP, kidney renal papillary cell carcinoma; LAML, acute myeloid leukaemia; LGG, brain lower-grade glioma; LUAD, lung adenocarcinoma; LUSC, lung squamous cell carcinoma; OV, ovarian serous cystadenocarcinoma; PAAD, pancreatic adenocarcinoma; PRAD, prostate adenocarcinoma; SKCM, skin cutaneous melanoma; STAD, stomach adenocarcinoma; THCA, thyroid carcinoma; UCEC, uterine corpus endometrial carcinoma; UCS, uterine carcinosarcoma. Figure 2: Concurrent ARID1A loss and PIK3CA activation leads to ovarian tumorigenesis in the mouse. ( a ) Plot of ARID1A and PIK3CA alterations across available TCGA data sets. Mutation or co-mutation frequencies are expressed as a percentage of all tumour samples for each cancer. A Fisher’s exact test was used to calculate the significance of association between ARID1A and PIK3CA mutations (* P value <0.05). ( b ) Genotyping scheme to detect CRE-deleted ( Arid1aΔ ) allele in tumour genomic DNA samples. RT–PCR was used to distinguish PIK3CA and transgenic (Gt)Rosa26Pik3ca *H1047R transcripts in tumour RNA samples. The H1047R mutation in (Gt)Rosa26Pik3ca *H1047R protects against MslI digest of amplified tumour cDNA. ( c ) ARID1A loss or (Gt)Rosa26Pik3ca *H1047R transcripts were detected in tumour RNA samples by RT–PCR. Significant differences based on the average normalized mRNA expression ±s.d. between replicates of a control liver sample and replicates of three independent tumour samples were calculated using a two-tailed Student’s t -test ( P values <0.05 were considered significant). ( d , e ) ARID1A expression is observed in cells throughout the normal uterus and ovary by IHC. ( e ) ARID1A is expressed in the OSE of normal ovaries (arrowhead). ( f ) ARID1A expression is not observed in the tumours. ( g ) P-AKT S473 levels are low in the normal uterus. ( h , i ) P-AKT S473 in the normal ovary is highest in the OSE ( h , arrowhead) and these levels are greatly increased in ovarian tumours ( i , arrowhead). Asterisk in e denotes an oocyte. All sections processed for IHC were lightly counterstained with methyl green. ( j , k ) Morbid Arid1a fl/fl ; (Gt)Rosa26Pik3ca *H1047R mouse at killing with haemorrhagic ascites (inset), primary ovarian tumour of moderate size and bilateral tumour metastases (arrowheads). ( l , m ) Morbid Arid1a fl/fl ; (Gt)Rosa26Pik3ca *H1047R mouse at killing with haemorrhagic ascites (inset), large primary ovarian tumour and no visible metastases. The mice shown in j – m were killed at 7 and 9 weeks post AdCRE, respectively, because of visible ascitic fluid burden. ( n , o ) Arid1a fl/+ ; (Gt)Rosa26Pik3ca *H1047R mice at 11 weeks post AdCRE showing no evidence for tumour formation. In k , m , dashed circles indicate primary ovarian tumour on injected ovary. In n , arrows denote the AdCRE-injected ovary. In k , m , o , asterisks denote the uninjected, control ovary. ACC, adrenocortical carcinoma; BLCA, bladder urothelial carcinoma; BRCA, breast invasive carcinoma; CESC, cervical squamous cell carcinoma and endocervical adenocarcinoma; COAD/READ, colon and rectum adenocarcinoma; GBM, glioblastoma multiforme; HNSC, head and neck squamous cell carcinoma; KICH, kidney chromophobe; KIRC, kidney renal clear-cell carcinoma; KIRP, kidney renal papillary cell carcinoma; LAML, acute myeloid leukaemia; LGG, brain lower-grade glioma; LUAD, lung adenocarcinoma; LUSC, lung squamous cell carcinoma; OV, ovarian serous cystadenocarcinoma; PAAD, pancreatic adenocarcinoma; PRAD, prostate adenocarcinoma; SKCM, skin cutaneous melanoma; STAD, stomach adenocarcinoma; THCA, thyroid carcinoma; UCEC, uterine corpus endometrial carcinoma; UCS, uterine carcinosarcoma. Full size image PIK3CA tumour mutations often result in an H1047R ‘hotspot’ substitution within the kinase domain, generating a catalytically active protein [34] . PIK3CA amplification also frequently occurs in EOC [30] . To investigate the effect of PIK3CA alterations on ovarian tumorigenesis, we used the CRE-inducible (Gt)Rosa26Pik3ca *H1047R allele [35] to drive PIK3CA H1047R expression from the Rosa26 locus. We observed multifocal sites of epithelial hyperplasia in the OSE of AdCRE-injected (Gt)Rosa26Pik3ca *H1047R mice, but no tumour formation ( Table 1 ). Intrabursal AdCRE induction of PIK3CA H1047R , under the control of the endogenous promoter, also led to OSE hyperplasia in the mouse [36] , suggesting that constitutive overexpression of PIK3CA H1047R from the Rosa26 locus does not further augment this process. Table 1 Ovarian tumorigenesis requires concurrent ARID1A loss and PIK3CA activation. Full size table We next evaluated the combinatorial effects of ARID1A loss and PIK3CA activation by performing AdCRE injections into the ovarian bursa of Arid1a fl/fl ; (Gt)Rosa26Pik3ca *H1047R mice. In stark contrast to the single mutants, Arid1a fl/fl ; (Gt)Rosa26Pik3ca *H1047R mice rapidly developed primary ovarian tumours and showed evidence of abdominal distension, warranting killing with a median latency period of 7.5 weeks post AdCRE injection ( Fig. 2j–m ). Evidence for tumour-specific ARID1A loss and PIK3CA H1047R expression or PI3K pathway activation was detected by PCR amplification of tumour complementary DNA (cDNA) or by tumour immunohistochemistry (IHC) for ARID1A and phosphorylation of AKT at serine 473 (P-AKT S473; Fig. 2b–i ). Increased morbidity coincided with the presentation of haemorrhagic ascites ( Fig. 2j,l ). Peritoneal metastases were detected in ~50% of the double mutants, often residing near the contralateral, uninjected ovary ( Fig. 2k , see Table 1 ). Distant metastases beyond the abdominal cavity were not evident on gross examination. We did not find evidence for genome instability in Arid1a fl/fl ; (Gt)Rosa26Pik3ca *H1047R tumour samples using mouse high-density SNP (single-nucleotide polymorphism) arrays ( Supplementary Fig. 2 ). ARID1A haploinsufficiency does not lead to tumour formation Several studies point to a gene dose-dependent role for ARID1A in tumour suppression given the high incidence of heterozygous tumour mutations in cancer [19] . To determine if an ARID1A haploinsufficiency coupled with PI3K pathway activation leads to ovarian cancer in our model, we performed AdCRE injections on Arid1a fl/+ ; (Gt)Rosa26Pik3ca *H1047R mice. OSE hyperplasia was observed in five out of the seven Arid1a fl/+ ; (Gt)Rosa26Pik3ca *H1047R mice, but evidence of tumour formation was not detected after the 11-week observation period, similar to the (Gt)Rosa26Pik3ca *H1047R only cohort ( Fig. 2n,o , see Table 1 ). These data are consistent with the observation that most OCCC tumours carrying heterozygous mutations in ARID1A show the loss of ARID1A immunoreactivity and support the notion that additional mechanisms lead to the loss of ARID1A protein expression in OCCC [18] , [37] . Thus, ARID1A likely follows the classical ‘two-hit’ model of tumour suppression in OCCC. Therapeutic PIK3CA inhibition prolongs animal survival We next sought to examine the role of continued PIK3CA activation in the progression of ARID1A-deficient ovarian tumours and determine whether therapeutic PIK3CA inhibition would inhibit tumour cell growth and improve animal survival. Primary EOC tumour cells were isolated from the exfoliated tumour cell aggregates present in ascites fluid of tumour-burdened Arid1a fl/fl ; (Gt)Rosa26Pik3ca *H1047R mice and subcultured using established methods ( Fig. 3a ). Isolated tumour cells displayed ARID1A loss and heightened PI3K signalling, as evidence by the loss of ARID1A immunoreactivity and increased P-AKT S473 levels compared with normal OSE cells ( Fig. 3b ). Administration of the pan-class I PI3K inhibitor, BKM120 (Buparlisib) led to a dose-dependent decrease in P-AKT S473 and concomitant reduction in tumour cell viability (IC 50 =0.96±0.25 μM; Fig. 3c,d ). We next administered chow-fed BKM120 to Arid1a fl/fl ; (Gt)Rosa26Pik3ca *H1047R mice for 3 weeks, starting at week 4 post AdCRE injection. The effectiveness of BKM120-dependent inhibition of PI3K signalling in chow-fed mice was accessed by tumour IHC for phosphorylation of the S6 ribosomal protein at serine 235/236 (P-S6; Fig. 3e ). BKM120 treatment led to reduced P-S6 levels and extended the median latency period by 3.5 weeks ( Fig. 3e,f ). These data indicate that therapeutic PI3K inhibition promotes animal survival by inhibiting tumour cell growth, thus providing strong rationale for the use of PI3K inhibitors in OCCC treatment. 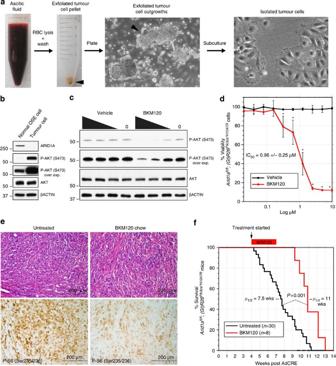Figure 3: Therapeutic PIK3CA inhibition promotes animal survival by reducing tumour cell viability. (a) Primary ascites-derived tumour cell isolation scheme. (b) Representative western blots to highlight the primary tumour cell validation scheme and demonstrate that ARID1A loss and heightened P-AKT S473 is observed in primaryArid1afl/fl;(Gt)Rosa26Pik3ca*H1047Rascitic tumour cells versus normal OSE cells. (c) Western blots of P-AKT S473 and total AKT levels inArid1afl/fl;(Gt)Rosa26Pik3ca*H1047Rascitic tumour cells grown in the presence 10, 1, 0.001 or 0 μM BKM120 or equivalent dilutions (v/v) of dimethylsulphoxide vehicle control for 48 h. (d) BKM120 treatment reduces tumour cell viability with a half-maximal inhibitory concentration (IC50) of 0.96±0.25 μM. Significant differences based on the average per cent inhibition ±s.d. of three independent tumour cell lines treated with BKM120- versus vehicle-treated cells were calculated using a two-tailed Student’st-test (*Pvalue <0.05). (e,f) Administration of chow-fed BKM120 reduces PI3K pathway activity, as shown by reduced P-S6 Ser235/236 levels, and extends theArid1afl/fl;(Gt)Rosa26Pik3ca*H1047Rmedian survival latency to 11 weeks. BKM120 treatment commenced 4 weeks after AdCRE injection. P-S6 Ser235/236 IHC was performed on tumour histological sections from three independent BKM120-treated or -untreated mice. (f) UntreatedArid1afl/fl;(Gt)Rosa26Pik3ca*H1047Rmice succumb to cancer with a median (μ1/2) latency of period of 7.5 weeks. Statistical differences in survival (BKM120 chow-fed versus untreated) were calculated using a log-rank test (Pvalues <0.05 were considered significant). Figure 3: Therapeutic PIK3CA inhibition promotes animal survival by reducing tumour cell viability. ( a ) Primary ascites-derived tumour cell isolation scheme. ( b ) Representative western blots to highlight the primary tumour cell validation scheme and demonstrate that ARID1A loss and heightened P-AKT S473 is observed in primary Arid1a fl/fl ; (Gt)Rosa26Pik3ca *H1047R ascitic tumour cells versus normal OSE cells. ( c ) Western blots of P-AKT S473 and total AKT levels in Arid1a fl/fl ; (Gt)Rosa26Pik3ca *H1047R ascitic tumour cells grown in the presence 10, 1, 0.001 or 0 μM BKM120 or equivalent dilutions (v/v) of dimethylsulphoxide vehicle control for 48 h. ( d ) BKM120 treatment reduces tumour cell viability with a half-maximal inhibitory concentration (IC 50 ) of 0.96±0.25 μM. Significant differences based on the average per cent inhibition ±s.d. of three independent tumour cell lines treated with BKM120- versus vehicle-treated cells were calculated using a two-tailed Student’s t -test (* P value <0.05). ( e , f ) Administration of chow-fed BKM120 reduces PI3K pathway activity, as shown by reduced P-S6 Ser235/236 levels, and extends the Arid1a fl/fl ; (Gt)Rosa26Pik3ca *H1047R median survival latency to 11 weeks. BKM120 treatment commenced 4 weeks after AdCRE injection. P-S6 Ser235/236 IHC was performed on tumour histological sections from three independent BKM120-treated or -untreated mice. ( f ) Untreated Arid1a fl/fl ; (Gt)Rosa26Pik3ca *H1047R mice succumb to cancer with a median ( μ 1/2 ) latency of period of 7.5 weeks. Statistical differences in survival (BKM120 chow-fed versus untreated) were calculated using a log-rank test ( P values <0.05 were considered significant). Full size image Mouse ovarian tumours manifest OCCC-like histopathology Cardinal histopathological features of human OCCC include cells with clear cytoplasm, stromal hyalinization, solid, papillary or tubulocystic tumour architectural patterns, and HNF1β immunoreactivity [38] . The ovarian tumours observed in Arid1a fl/fl ; (Gt)Rosa26Pik3ca *H1047R mice were predominately solid in appearance with some papillary areas ( Fig. 4a–d , see Table 1 ). Tubulocystic patterns were rarely observed ( Fig. 4e , see Table 1 ). Neoplastic cells with clear cytoplasm, prominent nucleoli and pleomorphic nuclei were observed in the tumours (see high magnification in Fig. 4a′–c′ ). Elongated spindle-shaped cells with finely vacuolated cytoplasm were observed embedded in hyalinized matrix. Solid clear-cell carcinomas were observed directly attached to the ovarian surface ( Fig. 4a ). We rarely observed tumour cells organized into bands of glandular epithelium with distinct borders, and, in general, the tumours appeared poorly differentiated and highly disorganized. Primary tumour masses ranged from ~100 mg to over 1 g ( Fig. 4j ). Differences in tumour size, metastatic potential or morbidity did not correlate with any particular histologic feature. 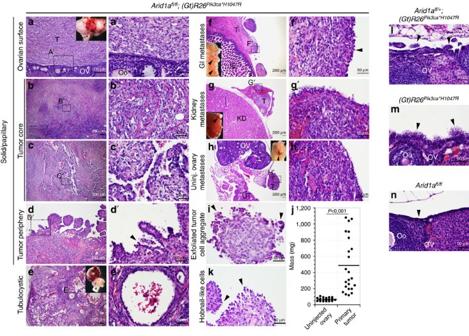Figure 4:Arid1afl/fl;(Gt)Rosa26Pik3ca*H1047Rovarian tumours manifest clear-cell-like histological features. (a–e) Haematoxylin and eosin (H&E)-stained sections of tumour architectural patterns observed in intrabursal AdCRE-injectedArid1afl/fl;(Gt)Rosa26Pik3ca*H1047Rmice. Whole-mount tumour images are shown inset ina,e. Asterisks denote the uterus. Dotted linea′demarcates the ovarian surface-tumour boundary. Arrowhead ind′denotes a hobnail cell. (f–h) H&E-stained sections ofArid1afl/fl;(Gt)Rosa26Pik3ca*H1047Rtumour metastases found on the surface of gastrointestinal tract (f), kidney (g) and uninjected, control ovary (h). (a′–h′) High-magnification images of regions demarcated by dashed boxes ina–h. (i) H&E-stained exfoliated tumour cell aggregate. (k) H&E-stained example of hobnail cells on the luminal surface of a tumour. Arrowheads ind′,f′,i,kdenote hobnail cells on tumour surface. (j) Dot plot of primary tumour mass compared with uninjected control ovary. Significant differences based on the average mass ±s.d. between tumours and matched uninjected ovaries were calculated using a two-tailed Student’st-test (Pvalues <0.05 were considered significant). (l–n) H&E-stained high-magnification images of the ovarian surface fromArid1afl/+;(Gt)Rosa26Pik3ca*H1047R,(Gt)Rosa26Pik3ca*H1047R, andArid1aflflmice. (m,n) OSE hyperplasia (arrowheads) is observed in(Gt)Rosa26Pik3ca*H1047RandArid1afl/+;(Gt)Rosa26Pik3ca*H1047Rmice. IE, intestinal epithelium; KD, kidney; Oo, oocyte; OV, ovary; T, tumour; UT, uterus. Figure 4: Arid1a fl/fl ; (Gt)Rosa26Pik3ca *H1047R ovarian tumours manifest clear-cell-like histological features. ( a – e ) Haematoxylin and eosin (H&E)-stained sections of tumour architectural patterns observed in intrabursal AdCRE-injected Arid1a fl/fl ; (Gt)Rosa26Pik3ca *H1047R mice. Whole-mount tumour images are shown inset in a , e . Asterisks denote the uterus. Dotted line a′ demarcates the ovarian surface-tumour boundary. Arrowhead in d′ denotes a hobnail cell. ( f – h ) H&E-stained sections of Arid1a fl/fl ; (Gt)Rosa26Pik3ca *H1047R tumour metastases found on the surface of gastrointestinal tract ( f ), kidney ( g ) and uninjected, control ovary ( h ). ( a′ – h′ ) High-magnification images of regions demarcated by dashed boxes in a – h . ( i ) H&E-stained exfoliated tumour cell aggregate. ( k ) H&E-stained example of hobnail cells on the luminal surface of a tumour. Arrowheads in d ′, f ′, i , k denote hobnail cells on tumour surface. ( j ) Dot plot of primary tumour mass compared with uninjected control ovary. Significant differences based on the average mass ±s.d. between tumours and matched uninjected ovaries were calculated using a two-tailed Student’s t -test ( P values <0.05 were considered significant). ( l – n ) H&E-stained high-magnification images of the ovarian surface from Arid1a fl/+ ; (Gt)Rosa26Pik3ca *H1047R , (Gt)Rosa26Pik3ca *H1047R , and Arid1a flfl mice. ( m , n ) OSE hyperplasia (arrowheads) is observed in (Gt)Rosa26Pik3ca *H1047R and Arid1a fl/+ ; (Gt)Rosa26Pik3ca *H1047R mice. IE, intestinal epithelium; KD, kidney; Oo, oocyte; OV, ovary; T, tumour; UT, uterus. Full size image In human OCCC, neoplastic cells that line the luminal spaces often assume a ‘hobnail’ appearance, which crudely resembles a nucleus standing on the tip of a cytoplasmic stalk. Hobnail cells were often observed on the tumour periphery in regions where tumour cell exfoliation into luminal regions was occurring ( Fig. 4d,i,k ). Exfoliated, metastatic tumour cell aggregates often consisted of hobnail-shaped cells organized around either clear-cell or hyalinized cores ( Fig. 4i ). OSE hyperplasia and small clumps of hobnail cells were evident on the ovarian surface as early as 1 week following AdCRE injection, with exfoliated tumour cell aggregates and clear-cell-like features apparent at 2 weeks ( Supplementary Fig. 3 ). The tumours were also positive for the human OCCC marker, HNF1β, by IHC ( Fig. 5b ). Thus, mouse ovarian tumours harbouring coexistent ARID1A–PIK3CA mutations share histopathological features with human OCCC. 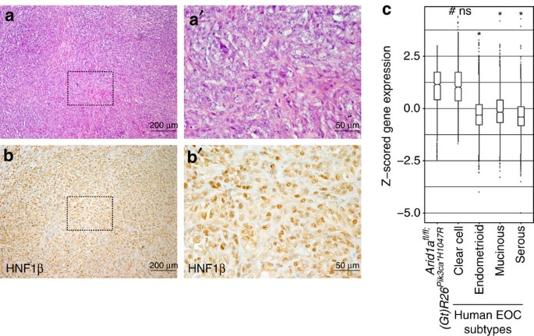Figure 5:Arid1afl/fl;(Gt)Rosa26Pik3ca*H1047Rovarian tumours and human OCCC share molecular characteristics. (a) Haematoxylin and eosin-stained image ofArid1afl/fl;(Gt)Rosa26Pik3ca*H1047Rtumour histology. (b) Near-adjacent histological section showing HNF1β immunoreactivity by IHC. (a′,b′) High-magnification images of regions demarcated by dashed boxes ina,b. (c) Box plots of normalized expression values of human OCCC discriminant genes (N=159) for all mouse tumour and human EOC subtype samples. Significant differences between the mouse tumours and each human histological EOC subtype were calculated using a Wilcoxon test (*significantPvalue of <0.05; #not significantPvalue=0.6). NS, not significant. Figure 5: Arid1a fl/fl ; (Gt)Rosa26Pik3ca *H1047R ovarian tumours and human OCCC share molecular characteristics. ( a ) Haematoxylin and eosin-stained image of Arid1a fl/fl ; (Gt)Rosa26Pik3ca *H1047R tumour histology. ( b ) Near-adjacent histological section showing HNF1β immunoreactivity by IHC. ( a′ , b′ ) High-magnification images of regions demarcated by dashed boxes in a , b . ( c ) Box plots of normalized expression values of human OCCC discriminant genes ( N =159) for all mouse tumour and human EOC subtype samples. Significant differences between the mouse tumours and each human histological EOC subtype were calculated using a Wilcoxon test (*significant P value of <0.05; #not significant P value=0.6). NS, not significant. Full size image Tumour gene expression supports a role for IL-6 in OCCC To further evaluate the relevance of our Arid1a fl/fl ; (Gt)Rosa26Pik3ca *H1047R ovarian tumour model to human OCCC, we performed a series of cross-species gene expression comparisons using a well-characterized gene expression data set containing all four human EOC subtypes [39] . Gene expression profiles of mouse primary tumour samples and matched normal (uninjected) ovaries were generated by microarray. Consistent with our genetic model, ARID1A and PIK3CA expression levels were inversely correlated in comparisons between tumour and normal ovary samples, with PIK3CA upregulation strongly correlated with ARID1A downregulation in the tumour samples ( Supplementary Fig. 4 ). We verified our microarray gene expression results by reverse transcription-PCR (RT–PCR) validation of KRAS, TFPI2, CDKN2A (P16), CDKN1A (P21), MUC16 (CA125) and VCAN expression ( Supplementary Fig. 5 ). We next identified all coordinately regulated genes in both mouse tumours and human OCCC, as compared with species-matched normal ovaries. In comparisons of both mouse and human data sets, the control ovary samples showed high levels of gene expression variation, suggesting tissue sampling differences or general interspecies-specific gene expression differences ( Supplementary Fig. 6 ). Focusing on those genes that remained unchanged in normal mouse and human ovaries, we identified 584 coordinately regulated genes (272 upregulated; 312 downregulated) in mouse and human tumours ( Supplementary Fig. 7 ). Mouse and human tumour gene expression patterns were enriched for genes involved in IL-6 signalling, immune system function, focal adhesion and regulation of the actin cytoskeleton, as compared with normal ovaries ( Supplementary Figs 6 and 7 ). Since many of the upregulated genes we identified in cross-species comparisons with normal ovaries are likely to be found in other EOC subtypes (for example, CA125) or generally found across most cancers, we next sought to identify an OCCC-specific gene signature for use in subtype-specific gene expression comparisons with the mouse tumours. To do this, we compiled a more refined ‘discriminant’ gene list for each subtype (for example, clear-cell versus all other EOC subtypes). We then compared the normalized raw expression values for each discriminant gene across all of the mouse tumour and human EOC samples. Using this analysis, we found that the gene expression patterns for mouse tumour and human OCCC samples were not statistically different ( P =0.6), suggesting that the OCCC-specific gene expression patterns are conserved between the two species ( Fig. 5c ). Several well-known markers of OCCC were identified as being highly expressed in the mouse tumours, including IL-6, STAT3, VCAN and HIF1α, further supporting a role for heightened IL-6 signalling in OCCC tumour pathogenesis [40] , [41] , [42] ( Fig. 6a ). 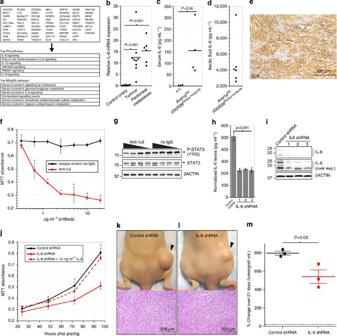Figure 6: Tumour-derived IL-6 promotes OCCC tumour cell growth and survival. (a) Top OCCC-specific genes in common between mouse and human tumours. Top six Ingenuity Pathway Analysis (IPA) and MSigDB (GSEA) predictions of the top upregulated genes are included. (b) RT–PCR validation of IL-6 expression in primary tumours and peritoneal metastases. Significant differences based on average normalized mRNA expression ±s.d. between peritoneal metastases or primary tumours and matched uninjected ovaries were calculated using a two-tailed Student’st-test. (c,d) Mouse IL-6 levels in the serum and ascitic fluidArid1afl/fl;(Gt)Rosa26Pik3ca*H1047Rmice, as measured by anti-IL-6 ELISAs. Significant differences based on the average protein concentration ±s.d. between wild-type versusArid1afl/fl;(Gt)Rosa26Pik3ca*H1047Rmice were calculated using a two-tailed Student’st-test. (e) IL-6 expression in anArid1afl/fl;(Gt)Rosa26Pik3ca*H1047Rtumour by IHC. (f) MTT absorbance values plotted with log antibody concentration (μg ml−1) for non-specific rat IgG-treated (control) or rat anti-mouse IL-6-treatedArid1afl/fl;(Gt)Rosa26Pik3ca*H1047Rascitic tumour cells after 96 h. of treatment. Plot represents the average absorbance value±s.d. for treatment performed on three independent cell lines. Significant differences between control- and anti-IL-6-treated cells were calculated using a two-tailed Student’st-test (*significantPvalue <0.05). (g) Primary ascitic tumour cells were treated 10, 1, 0.01 or 0 μg ml−1rat anti-mouse IL-6 or non-specific Rat IgG-treated (control). (h,i) IL-6 expression inArid1afl/fl;(Gt)Rosa26Pik3ca*H1047Rascitic tumour cells stably expressing control shRNAs or IL-6 shRNAs by ELISA and western blot. Each replicate represents in stable pool of IL-6 shRNA-expressing cells from three independently isolated tumour cell lines. Significant differences based on the average protein concentration ±s.d. between control versus IL-6 shRNA were calculated using a two-tailed Student’st-test. (j) MTT absorbance values plotted over time for control shRNA-, IL-6 shRNA- or IL-6 shRNA-expressing cells supplemented with 10 ng ml−1IL-6. Cells were plated at 2 × 10e4 cells ml−1at hour 0, then MTT measurements were taken every 24 h for a total of 96 h. Significant differences between control- and IL-6 shRNA-expressing cells were calculated using a two-tailed Student’st-test (*significantPvalue < 0.05). (k,l) Whole-mount images of control- and IL-6 shRNA tumorgrafts (arrowheads) on the right flank of nude mice and images of corresponding haematoxylin and eosin-stained tumorgraft sections. (m) Plot of growth rates for control- and IL-6 shRNA-expressing tumorgrafts over 21 days of measurement. Significant differences between control- and IL-6 shRNA tumorgraft growth rates were calculated using a two-tailed Student’st-test. OnlyPvalues <0.05 were considered significant. MTT, 3-(4,5-dimethylthiazol-2-yl)-2,5-diphenyltetrazolium bromide. Figure 6: Tumour-derived IL-6 promotes OCCC tumour cell growth and survival. ( a ) Top OCCC-specific genes in common between mouse and human tumours. Top six Ingenuity Pathway Analysis (IPA) and MSigDB (GSEA) predictions of the top upregulated genes are included. ( b ) RT–PCR validation of IL-6 expression in primary tumours and peritoneal metastases. Significant differences based on average normalized mRNA expression ±s.d. between peritoneal metastases or primary tumours and matched uninjected ovaries were calculated using a two-tailed Student’s t -test. ( c , d ) Mouse IL-6 levels in the serum and ascitic fluid Arid1a fl/fl ; (Gt)Rosa26Pik3ca *H1047R mice, as measured by anti-IL-6 ELISAs. Significant differences based on the average protein concentration ±s.d. between wild-type versus Arid1a fl/fl ; (Gt)Rosa26Pik3ca *H1047R mice were calculated using a two-tailed Student’s t -test. ( e ) IL-6 expression in an Arid1a fl/fl ; (Gt)Rosa26Pik3ca *H1047R tumour by IHC. ( f ) MTT absorbance values plotted with log antibody concentration (μg ml −1 ) for non-specific rat IgG-treated (control) or rat anti-mouse IL-6-treated Arid1a fl/fl ; (Gt)Rosa26Pik3ca *H1047R ascitic tumour cells after 96 h. of treatment. Plot represents the average absorbance value±s.d. for treatment performed on three independent cell lines. Significant differences between control- and anti-IL-6-treated cells were calculated using a two-tailed Student’s t -test (*significant P value <0.05). ( g ) Primary ascitic tumour cells were treated 10, 1, 0.01 or 0 μg ml −1 rat anti-mouse IL-6 or non-specific Rat IgG-treated (control). ( h , i ) IL-6 expression in Arid1a fl/fl ; (Gt)Rosa26Pik3ca *H1047R ascitic tumour cells stably expressing control shRNAs or IL-6 shRNAs by ELISA and western blot. Each replicate represents in stable pool of IL-6 shRNA-expressing cells from three independently isolated tumour cell lines. Significant differences based on the average protein concentration ±s.d. between control versus IL-6 shRNA were calculated using a two-tailed Student’s t -test. ( j ) MTT absorbance values plotted over time for control shRNA-, IL-6 shRNA- or IL-6 shRNA-expressing cells supplemented with 10 ng ml −1 IL-6. Cells were plated at 2 × 10e4 cells ml −1 at hour 0, then MTT measurements were taken every 24 h for a total of 96 h. Significant differences between control- and IL-6 shRNA-expressing cells were calculated using a two-tailed Student’s t -test (*significant P value < 0.05). ( k , l ) Whole-mount images of control- and IL-6 shRNA tumorgrafts (arrowheads) on the right flank of nude mice and images of corresponding haematoxylin and eosin-stained tumorgraft sections. ( m ) Plot of growth rates for control- and IL-6 shRNA-expressing tumorgrafts over 21 days of measurement. Significant differences between control- and IL-6 shRNA tumorgraft growth rates were calculated using a two-tailed Student’s t -test. Only P values <0.05 were considered significant. MTT, 3-(4,5-dimethylthiazol-2-yl)-2,5-diphenyltetrazolium bromide. Full size image To further assess the similarities between our genetic model and human OCCC, we compared the mouse tumour-specific gene expression profiles for our Arid1a fl/fl ; (Gt)Rosa26Pik3ca *H1047R mouse model to those recently reported for the Arid1a fl/fl ; Pten fl/fl mouse model by Guan et al . [26] , which is genetically similar endometrioid EOC. Both models relied on the intrabursal AdCRE injection method for mutation induction. We applied principal component analysis using the normalized expression values for all genes in the tumour data sets for each mouse model. We found that each tumour sample clustered based on the genotype or mutational pattern of the respective genetic model, with the exception of one Arid1a fl/fl ; Pten fl/fl tumour ( Supplementary Fig. 8 ). These findings are consistent with the marked phenotypic differences observed in our Arid1a fl/fl ; (Gt)Rosa26Pik3ca *H1047R tumours when compared with the phenotypes reported for Arid1a fl/fl ; Pten fl/fl tumours by Guan et al . [26] Autocrine IL-6 signalling promotes tumour cell growth IL-6 is an inflammatory cytokine that triggers JAK/STAT3 signalling and has prominent roles in tumour cell growth and differentiation [43] , [44] . High levels of circulating IL-6 in cancer patients are associated with a poor prognosis [43] , [44] . In addition to its increased expression in OCCC tumours, IL-6 has been detected in patient serum and tumour-derived cell lines, which has led to its proposed use as a therapeutic target in OCCC [40] , [41] , [42] . In support of our cross-species microarray comparisons, we verified IL-6 expression in primary tumours and peritoneal metastases of Arid1a fl/fl ; (Gt)Rosa26Pik3ca *H1047R mice by RT–PCR ( Fig. 6b ). We also observed high levels of secreted IL-6 in the body fluids of tumour-burdened mice, with >2,000 pg ml −1 of IL-6 in ascitic fluid aspirates ( Fig. 6c,d ). Consistent with this, strong IL-6 immunoreactivity was also observed in the mouse tumours by IHC ( Fig. 6e ). To understand the role of IL-6 in OCCC pathogenesis, we treated primary Arid1a fl/fl ; (Gt)Rosa26Pik3ca *H1047R mouse ascites-derived tumour cells, isolated as described above, with anti-IL-6-neutralizing antibodies. Anti-IL-6 treatment reduced the tumour cell viability and downregulated the phosphorylation of STAT3 at tyrosine 705 (P-STAT3 Y705), suggesting that autocrine IL-6-STAT3 signalling promotes tumour cell growth ( Fig. 6f,g ). Next we generated primary mouse tumour cell lines that stably express IL-6 short hairpin RNAs (shRNA) for use in tumour growth assays ( Fig. 6h,i ). IL-6 shRNA-expressing cells showed reduced growth rates in culture, and media supplementation with recombinant IL-6 restored the normal growth patterns of IL-6 shRNA-expressing cells ( Fig. 6j ). To further examine tumour cell autonomous roles for IL-6 in ovarian tumour cell growth, we grafted control shRNA- and IL-6 shRNA-expressing mouse tumour cells onto the flanks of immunodeficient nude mice. Remarkably, the ascitic tumour cell grafts were indistinguishable from the ovarian tumours with regards to histopathological features (for example, clear cytoplasm), despite being maintained in tissue culture and further grown under the skin of immunodeficient mice ( Fig. 6k,l ). The rate of tumorgraft growth for IL-6 shRNA-expressing cells was significantly less than control shRNA-expressing cells, further indicating that autocrine IL-6 signalling contributes to OCCC pathogenesis by promoting tumour cell growth ( Fig. 6m ). IL-6 induction requires coexistent ARID1A–PIK3CA mutations To determine if coexistent ARID1A–PIK3CA mutations are required for IL-6 induction, we utilized an AdCRE-inducible primary OSE cell culture model. IL-6 expression was measured following AdCRE infection of primary OSE cells isolated from mice carrying all mutant allele combinations. Loss of ARID1A or PIK3CA activation alone led to significant increases in IL-6 expression by RT–PCR and enzyme-linked immunosorbent assay (ELISA), and IL-6 induction was further enhanced when ARID1A and PIK3CA were co-mutated together in Arid1a fl/fl ; (Gt)Rosa26Pik3ca *H1047R cells ( Fig. 7a,b ). Consistent with this, P-STAT3 Y705 levels also correlated with similar increases in IL-6 activity in AdCRE-treated OSE cells ( Fig. 7c ). ARID1A loss in AdCRE-treated Arid1a fl/fl or Arid1a fl/fl ; (Gt)Rosa26Pik3ca *H1047R OSE cells did not further enhance PI3K pathway activity ( Fig. 7c ). We found that Arid1a fl/fl ; (Gt)Rosa26Pik3ca *H1047R OSE cell proliferation was suppressed by treatment with anti-IL-6-neutralizing antibodies following mutation induction with AdCRE, and that recombinant IL-6 enhances normal OSE cell proliferation and IL-6-STAT3 signalling, further suggesting that IL-6 is both necessary and sufficient for tumour cell growth ( Fig. 7d–f ). To determine if ARID1A is bound at the IL-6 promoter under repressed conditions, we performed a series of ARID1A chromatin immunoprecipitation (ChIP) experiments in primary OSE cells. We used Arid1a fl/fl ; (Gt)Rosa26Pik3ca *H1047R OSE cells for these experiments so that AdCRE-treated or ARID1A-depleted cells could be used as a control for ARID1A immunoprecipitation specificity. In AdControl-treated cells, increased ARID1A occupancy was observed at sites near the IL-6 promoter, but not at distal upstream or downstream sites ( Fig. 7g ). ARID1A occupancy at this site decreased in a manner consistent with ARID1A depletion following AdCRE infection. These data indicate that coexistent ARID1A–PIK3CA mutations lead to IL-6 upregulation. 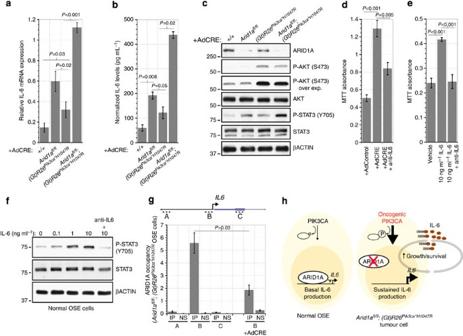Figure 7: Coexistent ARID1A–PIK3CA mutations induce IL-6 expression in a cooperative manner. (a) IL-6 mRNA expression in AdCRE-infected primary OSE cells carrying all allele combinations. (b) Normalized IL-6 ELISA measurements of AdCRE-infected primary OSE cells carrying all allele combinations. Significant differences based on the average normalized expression value ±s.d. among mutant allele combinations versus wild type were calculated using a two-tailed Student’st-test. (c) Western blot showing ARID1A, P-AKT S473, total AKT, P-STAT3 Y705 and total STAT3 levels in AdCRE-infected primary OSE cells carrying all allele combinations. AdCRE-infected wild-type cells served as controls. (d) MTT cell viability assay on primaryArid1afl/fl;(Gt)Rosa26Pik3ca*H1047ROSE cells treated with AdControl, AdCRE or AdCRE supplemented with 5 μg ml−1anti-IL-6 antibodies. (e) Treatment of normal (wild-type) primary OSE cells with vehicle (v/v), 10 ng ml−1IL-6 or 10 ng ml−1IL-6 supplemented with 5 μg ml−1anti-IL-6 antibodies. Significant differences based on the average MTT absorbance value ±s.d. between three independent replicates of AdControl- versus AdCRE-infected or vehicle- versus IL-6-treated cells were calculated using a two-tailed Student’st-test. (f) Western blot of normal primary OSE cells showing dose-dependent increases in P-STAT3 Y705 levels following IL-6 treatment. Co-treatment with 5 μg ml−1anti-IL-6 antibodies blocked P-STAT3 Y705 induction. (g) ARID1A occupancy at theIL-6locus was detected by ChIP using anti-ARID1A antibodies (denoted as IP) on crosslinked chromatin from AdControl- or AdCRE-infectedArid1afl/fl;(Gt)Rosa26Pik3ca*H1047Rprimary OSE cells. Non-specific isotype-matched antibodies (denoted as NS) were used in control ChIPs. ARID1A occupancy at theIL-6promoter (site or primer pairb) is reduced in ARID1A-depleted cells treated with AdCRE. Average per cent ChIP input ±s.d. represent data from experiments performed using three primary OSE cell isolations. Significant differences were calculated using a two-tailed Student’st-test. (h) Proposed model of IL-6 regulation by ARID1A and PIK3CA mutations in OCCC. OnlyPvalues <0.05 were considered significant. Figure 7: Coexistent ARID1A–PIK3CA mutations induce IL-6 expression in a cooperative manner. ( a ) IL-6 mRNA expression in AdCRE-infected primary OSE cells carrying all allele combinations. ( b ) Normalized IL-6 ELISA measurements of AdCRE-infected primary OSE cells carrying all allele combinations. Significant differences based on the average normalized expression value ±s.d. among mutant allele combinations versus wild type were calculated using a two-tailed Student’s t -test. ( c ) Western blot showing ARID1A, P-AKT S473, total AKT, P-STAT3 Y705 and total STAT3 levels in AdCRE-infected primary OSE cells carrying all allele combinations. AdCRE-infected wild-type cells served as controls. ( d ) MTT cell viability assay on primary Arid1a fl/fl ; (Gt)Rosa26Pik3ca *H1047R OSE cells treated with AdControl, AdCRE or AdCRE supplemented with 5 μg ml −1 anti-IL-6 antibodies. ( e ) Treatment of normal (wild-type) primary OSE cells with vehicle (v/v), 10 ng ml −1 IL-6 or 10 ng ml −1 IL-6 supplemented with 5 μg ml −1 anti-IL-6 antibodies. Significant differences based on the average MTT absorbance value ±s.d. between three independent replicates of AdControl- versus AdCRE-infected or vehicle- versus IL-6-treated cells were calculated using a two-tailed Student’s t -test. ( f ) Western blot of normal primary OSE cells showing dose-dependent increases in P-STAT3 Y705 levels following IL-6 treatment. Co-treatment with 5 μg ml −1 anti-IL-6 antibodies blocked P-STAT3 Y705 induction. ( g ) ARID1A occupancy at the IL-6 locus was detected by ChIP using anti-ARID1A antibodies (denoted as IP) on crosslinked chromatin from AdControl- or AdCRE-infected Arid1a fl/fl ; (Gt)Rosa26Pik3ca *H1047R primary OSE cells. Non-specific isotype-matched antibodies (denoted as NS) were used in control ChIPs. ARID1A occupancy at the IL-6 promoter (site or primer pair b ) is reduced in ARID1A-depleted cells treated with AdCRE. Average per cent ChIP input ±s.d. represent data from experiments performed using three primary OSE cell isolations. Significant differences were calculated using a two-tailed Student’s t -test. ( h ) Proposed model of IL-6 regulation by ARID1A and PIK3CA mutations in OCCC. Only P values <0.05 were considered significant. Full size image Our data support a genetic epistasis model wherein ARID1A and PIK3CA mutations cooperate and ovarian cancer can arise only when these genes are co-mutated in the mouse OSE. The short latency period, lack of copy-number variation and OCCC-like histological and molecular features we observed are also consistent with coexistent ARID1A – PIK3CA mutations being a major driver of OCCC in humans. Our results suggest that high levels of tumour cell-derived IL-6 are promoting tumour growth in OCCC. Indeed, the top pathway we identified in common between species is comprised of genes involved in this pathway, suggesting that IL-6-STAT3 signalling is inherent to OCCC biology. Hence, IL-6 serves as both a molecular marker and a prospective therapeutic target in OCCC. Therefore, anti-IL-6 antibody (Siltuximab) therapy may prove to be a safe and effective treatment strategy for OCCC patients. More broadly, our findings further demonstrate that the continued identification of tumour mutations (that is, TCGA projects) will allow us to identify potential functional relationships among recurrent mutational patterns or cancer pathways that would have otherwise gone unnoticed. The OSE-derived tumour phenotypes we observed in our Arid1a fl/fl ; (Gt)Rosa26Pik3ca *H1047R mouse model of OCCC greatly contrasted with those reported by Guan et al . [26] for Arid1a fl/fl ; Pten fl/fl mice. For example, all of the tumour-burdened Arid1a fl/fl ; (Gt)Rosa26Pik3ca *H1047R mice were morbid or succumbed to death within 3 months after AdCRE injection, whereas Guan et al . [26] reported tumours in a subset of Arid1a fl/fl ; Pten fl/fl mice after 6 months, indicating stark differences in tumour latency or survival. Molecular differences were evident in tumour gene expression comparisons between the two mouse models, as each gene expression data set parsed the majority of tumour samples based on its respective mutational pattern or genotype. These data point to potential functional differences between ARID1A–PIK3CA and ARID1A-PTEN mutational patterns in Type I EOCs and support the idea of a possible PI3K-AKT-mTOR-independent role for PTEN in endometrioid EOC [26] . Alternatively, it remains possible that clear-cell tumorigenesis is driven, in part, by an alternative AKT-independent mechanism downstream of oncogenic PIK3CA mutations [45] , [46] . Additional pharmacological studies targeting downstream effectors or alternative signalling pathway components will further address potential PI3K pathway-independent mechanisms of endometrioid versus clear-cell tumorigenesis. Several theories on the origins of OCCC have been proposed. Our data strongly suggest that the OSE harbours a cancer-prone cell population that gives rise to OCCC-like tumours in the mouse, which is consistent with the classical view of EOC pathogenesis. Nonetheless, our mouse model does not address the role of distal endometriotic explants or other putative precursor lesions in OCCC pathogenesis. Specifically targeting the ARID1A–PIK3CA mutational pattern to other tumour-prone epithelia within the Müllerian duct system would add relevance to our findings and help to further clarify the origins of EOC. An improved set of inducible CRE alleles would facilitate these experiments. Inflammation of coelomic epithelial cell derivatives in the female reproductive tract is thought to be a major contributor to malignant transformation in endometriosis-associated EOC, like OCCC [5] , [47] . Accordingly, inflammatory mediators, aberrant immune modulation or irregular reproductive hormone levels are thought to play a major role in malignant transformation [5] , [47] . Inflammatory cytokine signalling pathways, like IL-6, may be part of the natural inflammatory repair process accompanying each ovarian and menstrual cycle that, when left unchecked, promotes unregulated epithelial cell growth. In support of this, our data demonstrate that OSE cells are competent to respond to and upregulate IL-6. Therefore, the incomplete resolution of epithelial cell inflammation during these repair processes may represent a common mechanism underlying OCCC tumorigenesis, irrespective of mutational pattern. The identification of IL-6 as a physiological target of ARID1A tumour-suppressor activity in our OCCC tumour model raises many important questions regarding the role of ARID1A-containing SWI/SNF complexes in normal coelomic epithelial cell homeostasis. Indeed, ARID1A mutations have been identified in a wide variety of cancers originating from coelomic epithelial derivatives throughout the gynaecologic tract. Moreover, loss of ARID1A immunoreactivity is observed in endometriosis, a disease intimately associated with inflammation [48] , [49] , [50] . Endometriosis is also characterized by increased IL-6 expression, but the relationship between ARID1A loss and IL-6 upregulation in endometrial tissue is unknown [51] , [52] . Thus, ARID1A may regulate coelomic epithelial cell homeostasis and prevent tumorigenic conversion by negatively regulating the inflammatory programs required for normal tissue repair during the female reproductive cycle. It will be interesting to know if reproductive hormones influence ARID1A activity in this regard. Additional work on the propensity of ARID1A mutant epithelial cells to undergo malignant transformation in response to inflammatory ‘insults’ or the role of key inflammatory response pathways in this process will be required to address these hypotheses. Thus, the loss of ARID1A-containing SWI/SNF complexes might expose the ‘darker,’ pro-tumorigenic side of inflammation. How do oncogenic PI3K signalling mutations contribute to this process or lead to increased IL-6 expression? Positive regulators of IL-6 include JAK/STAT, PI3K, EGFR/HER2, RAS/RAF/MEK, TNF/TLR/IL1 or RAS/ERK oncogenic pathways and AP-1, SP1, NF-κB, C/EBP, STAT3, and CREB transcription factors [53] . IL-6-mediated JAK/STAT activation can further promote IL-6 transcription [53] . We propose that oncogenic PIK3CA H1047R mutations act like inflammatory ‘insults’ and drive the signalling loop that sustains high levels of IL-6 production in the absence of negative regulation by ARID1A ( Fig. 7h ). Additional studies focusing on the intricacies of this feed-forward signalling loop and the potential crosstalk mechanisms occurring among the various pathways that sustain it will further explain why coexistent ARID1A – PIK3CA mutations are found in a wide variety of human cancers. Generation of the Arid1a conditional mouse allele The Arid1a fl conditional mutant mouse allele was engineered using the bacterial artificial chromosome recombineering methods developed by Liu et al . [54] Correctly targeted mouse embryonic stem cell clones were identified by Southern blotting. The Neo selection cassette used for targeting was removed by FLP-mediated recombination [54] . Targeted embryonic stem cells were injected into C57Bl6 blastocysts and implanted into pseudopregnant females. Germline animals were detected by coat colour and PCR confirmation of tail DNA samples. AdCRE-mediated genetic recombination in the ovary To induce genetic recombination in the OSE, we employed a modified version of the ex vivo Adenovirus CRE (AdCRE) intrabursal delivery method [7] , [29] . In brief, AdCRE particles (obtained from the University of Iowa Gene Transfer Core) were diluted in sterile 1 × Dulbecco’s PBS (dPBS) containing 8 μg ml −1 polybrene. Deeply anaesthetized 8–10-week-old mice were given a single 5 μl injection of AdCRE particles (2.5 × 10 7 plaque-forming units or p.f.u.) into the right ovarian bursal cavity of the surgically exposed ovary using a sterile 31-gauge needle. Immediately following AdCRE injection, the surgically excised ovaries were washed with sterile 1 × dPBS and placed back into the abdominal cavity. The surgeries were performed on multiple occasions. Age- and genotype-matched, non-littermate animals were randomized before AdCRE injection. The surgeon was blinded to the genotypes before surgery and AdCRE injection. All surgical procedures were performed in accordance with protocols approved by the University of North Carolina at Chapel Hill Institutional Animal Care and Use Committee. Mouse husbandry and genotyping All mice were maintained on an outbred (random) genetic background using CD-1 mice (Charles River). (Gt)ROSA26 Pik3ca*H1047R and Sox2CRE alleles were purchased from the Jackson Laboratory and identified by PCR using published methods [28] , [35] . Arid1a +/+ ; Arid1a fl/+ ; Arid1a fl/fl alleles were distinguished by PCR using the following primer set: (F) 5′- CTAGGTGGAAGGTAGCTGACTGA -3′; (R) 5′- TACACGGAGTCAGGCTGAGC -3′. Combining the forward primer (from above) with the following reverse primer amplifies the CRE-excised allele: (R) 5′- AGAGTAACTAATAACTGCTGGAGGATG -3′. PCR products were resolved by 2% Tris-Borate-EDTA agarose gel electrophoresis. End points were palpable tumours (>1.5 cm 3 ), visible haemorrhagic ascites or severe abdominal distension, and signs of severe illness, such as dehydration, hunching, ruffled fur, signs of infection or non-responsiveness. Sample sizes within each genotype were chosen based on the proportions of animals with tumours and/or survival between each experimental group or a Kaplan–Meier log-rank test for survival differences. Whole-mount live-animal luminescent imaging was performed using the IVIS Optical System and reagents (Perkin Elmer) according to the manufacturer’s instructions. Whole-mount images of mice or necropsies were acquired using a Canon PowerShot SD1100 IS digital camera and a tabletop tripod. Whole-mount tumour specimens were imaged on a Leica MZ FLIII stereomicroscope using a DS Ri1 digital camera (Nikon). All mice were maintained at the University of North Carolina at Chapel Hill, Animal Facility using standard techniques in accordance with protocols approved by the University of North Carolina at Chapel Hill Institutional Animal Care and Use Committee. In vivo drug treatments The pan-PI3K inhibitor, BKM120 (Novartis) was milled by Research Diets using a vehicle- or carrier-free formulation similar to standard husbandry diets and dosed at 40 mg kg −1 based on the average daily oral consumption of a mouse [55] , [56] , [57] . AdCRE-injected animals were randomized before drug treatment. Control or untreated mice were given a standard husbandry diet. All drug treatments were performed in accordance with protocols approved by the University of North Carolina at Chapel Hill Institutional Animal Care and Use Committee. Reverse transcription-PCR Total RNA was extracted from pulverized tumour samples or ovarian epithelial cells using the TRIzol method (Invitrogen), followed by a RNA cleanup step and on-column DNA digestion using the RNAeasy mini prep kit (Qiagen) according to the manufacturers’ instructions. To analyse ARID1A and (Gt)Rosa26 Pik3ca*H1047R gene transcript levels, real-time quantitative PCR was performed using Ssofast PCR master mix (Biorad) and a CFX96 thermocycler (Biorad) with the following gene-specific primers: ARID1A (F) 5′- CTGAAGGACAAAGGTGACT -3′, ARID1A (R) 5′- CACAACTGCGAACTTCTC -3′; R26exon1 (F) 5′- CTAGGTAGGGGATCGGGACTCT -3′, PIK3CAcDNA (R) 5′- AATTTCTCGATTGAGGATCTTTTCT -3′ (ref. 35 ). The following gene-specific primers were used to validate the microarray expression data: KRAS (F) 5′- AGAGGAGTACAGTGCAATGAGG -3′, KRAS (R) 5′- AGGCACATCTTCAGAGTCCTTT -3′; TFPI2 (F) 5′- AAGGGCTTGTGTGAACCACG -3′, (R) 5′- CCACCACAGCCAGTATAGGTG -3′; CDKN1A (F) 5′- ATCCAGACATTCAGAGCCACAG -3′, (R) 5′- ACGAAGTCAAAGTTCCACCGT -3′; CDKN2A (F) 5′- GCTTCTCACCTCGCTTGTCA -3′, (R) 5′- AGTGACCAAGAACCTGCGAC -3′; MUC16 (F) 5′- CTCATCTGCTTGGCGGTACT -3′; (R) 5′- GAACCCTGCTAGGGAAGAGC -3′; VCAN (F) 5′- GAAGGGAACAGTTGCTTGCG -3′, (R) 5′- TTAGGCATTGCCCATCTCCC -3′; IL-6 (F) 5′- CACTTCACAAGTCGGAGGCT -3′, (R) 5′- CTGCAAGTGCATCATCGTTGT -3′. The expression was calculated from three independent experiments using ΔΔ C t methods. Expression levels were normalized to βACTIN . Statistical differences were detected using a two-tailed Student’s t -test. The following H1047 spanning PCR primer pair was used to distinguish endogenous PIK3CA from Rosa26 -derived, PIK3CA H1047R gene transcripts: (F) 5′- TTCAATGATGCTTGGCTCTG -3′; (R) 5′- CTGCTTGATGGTGTGGAAGA -3′. The PCR products were digested with MslI and resolved by 2% Tris-Borate-EDTA agarose gel electrophoresis. Western blotting Western blots were performed using the following antibody dilutions and standard chemiluminescent detection methods or Li-COR Bioscience Odyssey fluorescent western blotting reagents: 1:1,000 ARID1A (A301-041A, Bethyl Labs,), 1:500 IL-6 (ab6672, Abcam), 1:1,000 Phospho-AKT Ser473 (4060, Cell Signaling), 1:1,000 AKT (4691, Cell Signaling), 1:100 STAT3 (sc-482, Santa Cruz Biotechnology), 1:1,000 Phospho-STAT3 Tyr705 (9145, Cell Signaling) and 1:5,000 βACTIN (Abcam). Membranes were blocked in 1 × PBS supplemented with 5% (w/v) non-fat dry milk (Blotto A) or 1 × Tris-buffered saline (pH 7.6) supplemented with 5% (w/v) bovine serum albumin (BSA). Primary antibody incubations were performed in 1 × PBS supplemented with 1% (w/v) non-fat dry milk, 1% (w/v) BSA and 0.05% (v/v) Tween-20 (Blotto B) or 1 × Tris-buffered saline (pH 7.6) supplemented with 5% (w/v) BSA. Western blot images have been cropped for presentation. Full-size western blot images with antibody dilutions and blocking buffer conditions are presented in Supplementary Figs 9 and 10 . Enzyme-linked immunosorbent assay IL-6 ELISAs were performed using the OptEIA mouse IL-6 kit reagents (BD Bioscience) according to the manufacturer’s instructions. ELISA measurements were normalized to total cellular protein. Copy-number and TCGA computational analyses Tumour and matched control DNA samples were processed for hybridization on the high-density Mouse Universal Genotyping SNP Array (MegaMUGA, Neogen) using published methods [58] . Copy-number analysis was performed using ASCAT [59] . ARID1A and/or PIK3CA TCGA mutation frequency was identified by querying the cBioPortal on 2014-10-21 using the R API [60] , [61] . Microarray and cross-species gene expression comparisons Total RNA was isolated from nine primary tumour specimens and nine matched normal (uninjected) ovaries as described above. Total RNA (250 ng) was used to synthesize fragmented and labelled sense-strand cDNA and hybridize onto Affymetrix Mouse Gene 2.1 ST peg plate arrays. The mouse data were uploaded to the Gene Expression Omnibus (GEO) under the accession number: GSE57380 . Affymetrix CEL files were normalized using the Robust Multichip Average normalization method [62] . Expression changes (tumour versus control ovary) were determined using Linear Models for Microarray Data Analysis [63] or Significance Analysis of Microarray analysis [64] . Probes with a false discovery rate of 0% were considered statistically significant. For mouse–human cross-species comparisons, expression data for human OCCC and normal ovaries were downloaded from GEO under the accession number GSE6008 (ref. 39 ). Heat maps and dendrograms were generated with Java TreeView or R (www.R-project.org). Histological subtype-specific gene signatures were derived by first identifying differentially expressed genes between human normal tissue and cancer tissue in GSE6008. Next, differentially expressed genes were identified comparing each histological subtype to all other histological subtypes. We considered only upregulated genes, and any genes that were upregulated in both the tumour versus normal comparison and in a particular subtype were removed because these are not specific to a histological subtype and may reflect generic pan-cancer gene expression patterns. To compare human and mouse samples from these gene sets, we first determined Z -scores for each gene within the mouse or human. We combined these Z -scores and Z -scored the combined data using all human and mouse tumour samples in GSE6008 and this study. Pathways analysis was performed using the GSEA Molecular Signatures Database (MSigDB) [65] , [66] or Ingenuity Pathway Analysis (Qiagen). Ascites-derived tumour cell and OSE cell culture Primary ascites-derived ovarian tumour cells were isolated and grown as previously described [67] . To facilitate complete red blood cell lysis, the cell isolates were incubated and washed in deionized H 2 O before resuspension in growth medium. Mouse OSE cells were isolated and cultured as previously described [68] . To induce CRE-mediated recombination in OSE cells, the cells were infected with AdCRE or AdControl particles (obtained from the University of Iowa Gene Transfer Core) at an MOI of 200 for 2 h in serum-free media. Infected OSE cells were then placed in normal growth medium and allowed to recover for 3 days before further manipulation. BKM120 (Chemitek), low-endotoxin rat anti-mouse IL-6-neutralization antibody (R&D Systems, MAB406), non-specific rat IgG 1 isotype control antibody (R&D Systems, MAB005) or recombinant mouse IL-6 protein (R&D Systems, 406-ML-005) were reconstituted according to the manufacturers’ instructions and used as described in the text. For all antibody neutralization experiments, the cells were refed daily with the appropriate concentrations of antibody. Primary ascites-derived ovarian tumour cells were stably transduced with Mission pLKO.1-puro IL-6 shRNA (Hairpin sequence: 5′- CCGGCCAGAGTCCTTCAGAGAGATACTCGAGTATCTCTCTGAAGGACTCTGGTTTTTG -3′) (Sigma, TRCN0000067551) or non-target control shRNA (Sigma, SHC016V) Lentiviral transduction particles according to the manufacturers’ instructions. The MTT assay kit (Roche) was used to measure cell viability. Ascites-derived tumour cells and OSE cells were passaged using Accutase (Invitrogen). Half-maximal inhibitory concentrations (IC 50 ) were calculated by curve-fitting using Kaleidagraph software (Synergy). Tumour grafts Primary ascites-derived ovarian tumour cells expressing control- or IL-6 shRNAs were harvested by Accutase digestion and washed in 1 × dPBS. The cells were then injected subcutaneously into the right flanks of immunodeficient mice at a concentration of 5 × 10e7 cells ml −1 in a 1:1 (v/v) solution of 1 × dPBS and Cultrex basement membrane extract (3432-005-01, Trevigen). Tumour graft volumes were calculated using biweekly caliper-based measurements and growth rates were based on these volumetric measurements. All tumour grafts were performed in accordance with protocols approved by the University of North Carolina at Chapel Hill Institutional Animal Care and Use Committee. Histology and IHC For indirect IHC of slides, 10% neutral-buffered formalin-fixed paraffin sections were processed for heat-based antigen unmasking in 10 mM sodium citrate (pH 6.0). Sections were incubated with the following antibody dilutions: 1:50 ARID1A (Clone PSG3, sc-32761, Santa Cruz Biotechnology), 1:100 Cytokeratin 8 (TROMAI, DSHB), 1:50 phospho-AKT Ser473 (4060, Cell Signaling), 1:50 phospho-S6 Ribosomal Protein Ser235/236 (4858, Cell Signaling), 1:100 HNF1β (sc-7411, Santa Cruz Biotechnology) or 1:400 IL-6 (ab6672, Abcam). Vectastain Mouse-on-Mouse blocking reagents (Vector Labs) were used for ARID1A IHC. SignalStain antibody diluent (8112, Cell Signaling) and SignalSlide AKT controls (8115, Cell Signaling) were used for phospho-AKT Ser473 and phospho-S6 Ribosomal Protein Ser235/236 IHC. Secondary detection was performed using Vectastain ABC System reagents (Vector Labs). Sections processed for IHC were lightly counterstained with Haematoxylin QS or Methyl Green (Vector Labs). Routine haematoxylin and eosin staining of sections was performed by University of North Carolina, Lineberger Cancer Center, Animal Histopathology Core. Histological tumour assessments were reviewed by a UNC animal pathologist. Histological sections were analysed and photographed on an Olympus BX51 microscope using bright-field optics and a DP series digital camera (Olympus). Chromatin immunoprecipitation Primary OSE cells were fixed in growth media containing 1% methanol-free formaldehyde (Pierce) for 10 min at room temperature. The cells were washed twice with 1 × dPBS and then swelled in cell lysis buffer (5 mM Tris-Cl (pH 8.0); 85 mM KCl; 1% IGEPAL CA-630) for 10 min on ice. Swollen cells were homogenized (20 strokes) with a B-type dounce homogenizer on ice to facilitate nuclei release. Isolated nuclei corresponding to 1 × 10e7 cell equivalents per 500 μl of nuclear lysis buffer (50 mM Tris-Cl (pH 8.0), 10 mM EDTA and 0.3% SDS) and then sonicated using a water bath-cooled Diagenode Biorupter sonicator and 1.5 ml TPX microtubes (200 μl sample volume per tube) to an average DNA length between 300 and 700 bp. Chromatin concentrations were determined using a BCA protein assay kit (Pierce). Chromatin samples were diluted to 300 μg per 200 μl of nuclear lysis buffer and then cleared by centrifugation at 10,000 g . Precleared chromatin samples (200 μl each) were added to 800 μl (1:5 dilution) of ChIP dilution buffer (50 mM Tris-Cl (pH 7.5); 150 mM NaCl; 5 mM EDTA; 0.5% IGEPAL CA-630; 1% TX-100) and incubated with 10 μg of prebound ARID1A (Clone PSG3, 04-080, Millipore) Protein G dynal beads (Invitrogen) overnight at 4 °C. The Protein G dynal bead-anti-ARID1A immune conjugates were washed twice with 1 ml ChIP dilution buffer, three times with 1 ml ChIP dilution buffer supplemented with 500 mM NaCl, twice with 1 ml ChIP dilution buffer, followed by a final wash in 1 ml low-salt TE buffer (10 mM Tris-Cl (pH 8.0); 1 mM EDTA; 50 mM NaCl). The immunoprecipitated samples were eluted in 100 μl of elution buffer (50 mM NaHCO 3 ; 1% SDS) at 62 °C for 20 min. using an Eppendorf tube mixer. The crosslinks were reversed by adding NaCl to a final concentration of 0.2 M followed by an overnight incubation at 65 °C. The samples were then deproteinated with Proteinase K and purified using the ChIP DNA Clean & Concentrator kit (Zymo Research) according to the manufacturer’s instructions. Real-time quantitative PCR using Ssofast PCR master mix (Biorad) and a CFX96 thermocycler (Biorad) was performed using the following gene-specific primer pairs: (IL-6, Site A) 5′- GCAACTCTCACAGAGACTAAAGG -3′, 5′- GGACAACAGACAGTAATGTTGC -3′ (ref. 69 ); (IL-6, Site B) 5′- CTAGCCTCAAGGATGACTTAAGC -3′, 5′- CTATCGTTCTTGGTGGGCTCCAGAGC -3′ (ref. 70 ); (IL-6, Site C) 5′- GCCTTCTTGGGACTGATGCT -3′, 5′- GACAGGTCTGTTGGGAGTGG -3′. Data from three independent primary OSE cell isolations were averaged and plotted as a percentage of the total input. How to cite this article: Chandler, R. L. et al . Coexistent ARID1A–PIK3CA mutations promote ovarian clear-cell tumorigenesis through pro-tumorigenic inflammatory cytokine signalling. Nat. Commun. 6:6118 doi: 10.1038/ncomms7118 (2015). Accession codes : Microarray gene expression data sets generated in this study were deposited in the Gene Expression Omnibus (GEO) repository under the accession code GSE57380 .